Iridium-based double perovskites for efficient water oxidation in acid media The development of active, cost-effective and stable oxygen-evolving catalysts is one of the major challenges for solar-to-fuel conversion towards sustainable energy generation. Iridium oxide exhibits the best available compromise between catalytic activity and stability in acid media, but it is prohibitively expensive for large-scale applications. Therefore, preparing oxygen-evolving catalysts with lower amounts of the scarce but active and stable iridium is an attractive avenue to overcome this economical constraint. Here we report on a class of oxygen-evolving catalysts based on iridium double perovskites which contain 32 wt% less iridium than IrO 2 and yet exhibit a more than threefold higher activity in acid media. According to recently suggested benchmarking criteria, the iridium double perovskites are the most active catalysts for oxygen evolution in acid media reported until now, to the best of our knowledge, and exhibit similar stability to IrO 2 . (Photo-)electrochemical generation of fuels is a promising way to store renewable energy. However, large-scale electrochemical fuel generation is limited by the slow kinetics of the anode reaction (oxygen evolution reaction, OER) [1] . An active, stable and cost-effective OER catalyst compatible with the working conditions required for high-rate fuel production in polymer electrolyte membrane (PEM) electrolysers is still lacking [2] . The best available compromise between OER activity and stability at the moment is iridium oxide IrO 2 (refs 3 , 4 , 5 ), but it contains a large amount of iridium (one of the rarest elements on earth), making IrO 2 unsuitable for large-scale applications. Consequently, the development of OER catalysts with smaller amounts of iridium metal is a requirement towards cost-effective multi-MW solar fuel generation using PEM electrolysers, especially in combination with iridium recycling [6] , [7] . Complex iridium-based oxides (for example, perovskites, pyrochlores and fluorite-like compounds) are good alternatives to reduce the usage of the noble metal in the development of active and stable OER catalysts, by diluting iridium in a framework of less expensive materials. This alternative was explored by Kortenaar et al . [8] , who reported 12 iridium-based compounds with different crystal structures that exhibit from moderate to high OER catalytic activity in strong alkaline media (45% KOH). More recently, the group of Suntivich [9] reported that the SrIrO 3 simple perovskite exhibits higher OER activity than iridium oxide in alkaline media (0.1 M KOH). Since iridium-based OER catalysts are well suited to work in the acid environment of PEM electrolysers, this work explores the versatility of complex oxides to develop a class of catalysts for the OER in acid media. We report a family of catalysts based on iridium double perovskites, which contain three times less iridium and yet exhibit a more than threefold higher activity per cm 2 of real surface area (see Methods for details) for OER in acid media compared with IrO 2 , with similar stability. We show that these compounds are the most active catalysts for OER in acid media reported to date, to the best of our knowledge, according to recently suggested benchmarking criteria [10] . OER activity of the iridium-based double perovskites Double perovskites (DPs) are compounds with the generic formula A 2 BB′ O 6 , with A denoting a large cation and B and B′ smaller cations. The crystal structure of the ideal DP is depicted schematically in Fig. 1a (ref. 11 ). A wide range of compounds can be prepared by different combinations of A , B and B′ cations, which allows fine tuning of the DPs. The activity (measured as the current density) towards OER in 0.1 M HClO 4 (pH=1) was studied for Ba 2 MIrO 6 DPs, with M=Y, La, Ce, Pr, Nd and Tb. The electrodes were prepared by drop-casting an ethanol-based ink of the DPs on the gold disk of a rotating ring-disk assembly and the electrochemical experiments were carried out under rotating conditions (see Methods for further details). The structure of the Ir DPs was verified by powder X-ray diffraction (XRD) and the patterns obtained agree with those reported in the literature [12] , [13] , [14] ( Supplementary Fig. 1 ). 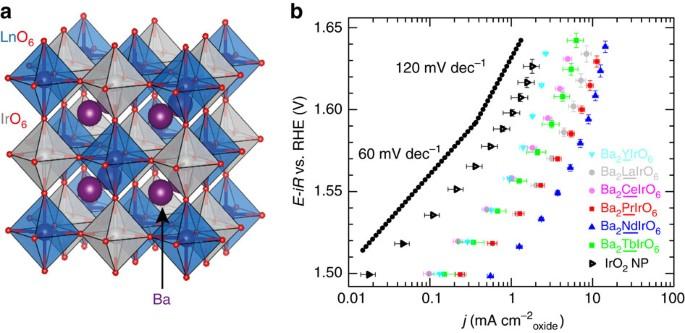Figure 1: Crystal structure and OER activity of the double perovskites. (a) Crystal structure of a generic Ba2MIrO6DP. (b) OER activity in 0.1 M HClO4of Ba2MIrO6, M=Y, La, Ce, Pr, Nd, Tb, compared with the benchmark activity of IrO2nanoparticles; the dotted lines show Tafel slopes of 60 and 120 mV per decade, to guide the eye. Measurements performed under steady-state conditions. The values in the plot are the average of three independent measurements and the error bars correspond to the s.d. Figure 1b summarizes the measured catalytic activities in the form of Tafel plots and compares the activity with IrO 2 nanoparticles that have been reported as the activity benchmark for OER in acid media [10] . The OER activity of the IrO 2 nanoparticles compares well with the values reported previously for similar nanoparticles [10] , [15] . Figure 1: Crystal structure and OER activity of the double perovskites. ( a ) Crystal structure of a generic Ba 2 MIrO 6 DP. ( b ) OER activity in 0.1 M HClO 4 of Ba 2 MIrO 6 , M=Y, La, Ce, Pr, Nd, Tb, compared with the benchmark activity of IrO 2 nanoparticles; the dotted lines show Tafel slopes of 60 and 120 mV per decade, to guide the eye. Measurements performed under steady-state conditions. The values in the plot are the average of three independent measurements and the error bars correspond to the s.d. Full size image All Ir DPs show a more than threefold higher activity per cm 2 of real surface area towards OER compared with the benchmarking IrO 2 nanoparticles. The surface area was calculated from pseudocapacitance measurements (see Methods for details). The OER activity depends on the cation in the B-site, in the order Ce≈Tb≈Y<La≈Pr<Nd. We note that we compare the intrinsic activity of the Ir DPs and the IrO 2 nanoparticles on the basis of the electrochemically active surface area. This intrinsic activity may be influenced by particle size [16] . Our Ir DPs are rather large ( ∼ 1 μm, see below) so it is to be expected that further activity adjustments may result from developing synthesis procedures yielding smaller particles. In addition to particle size, pH is an important parameter in activity comparisons. While Fig. 1b applies to pH=1 as we are primarily interested in the OER activity in acid media, it is well known that many oxides active for OER exhibit strongly pH-dependent reactivities [17] , [18] . Both the IrO 2 nanoparticles and the iridium-based DPs show two values for the Tafel slope, ca. 60 mV per decade between 1.5 and 1.6 V and 120 mV per decade above 1.6 V (numerical values are given in Supplementary Table 1 ). This feature has been reported previously for IrO 2 and was explained by a change in the mechanism for OH − adsorption, which is thought to be the rate-determining step for OER on IrO 2 (refs 19 , 20 ). We note, however, that the Tafel slope measured at high potentials for Ba 2 YIrO 6 (196+23 mV per decade) markedly deviates from the values for the other Ir DPs (ca. 120 mV per decade). We also measured the Faradaic efficiency of Ba 2 PrIrO 6 towards OER in 0.1 M HClO 4 in a rotating ring-disk electrode (RRDE) configuration ( Supplementary Fig. 2 ). It shows that Ba 2 PrIrO 6 has an efficiency towards water oxidation higher than 90% at 1.50 V ( η =0.27 V). The decrease in Faradaic efficiency with more anodic electrode potential is explained by the large current for OER above 1.6 V, leading to the formation of oxygen bubbles that reduce the detection efficiency on the ring. Stability of the Ir DPs under OER conditions The electrochemical stability of the Ir DPs was evaluated by galvanostatic electrolysis, in a manner similar to the approach reported by the JCAP group [10] . 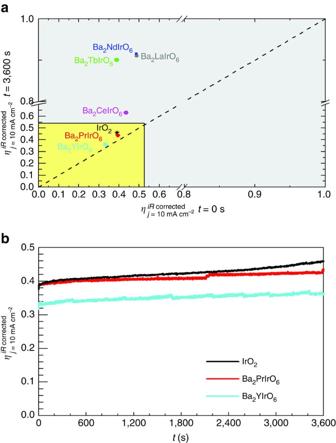Figure 2: Stability of the double perovskites under OER conditions. (a) OER overpotential measured on the Ir DPs after 1 h of galvanostatic electrolysis plotted as a function of the initial overpotential. (b) Evolution of the OER overpotential on Ba2PrIrO6, Ba2YIrO6DPs and IrO2nanoparticles during 1 h of galvanostatic electrolysis. Figure 2a summarizes the results obtained from these experiments. The stability of IrO 2 nanoparticles is presented for comparison. The diagonal dashed line represents the expected response of a stable catalyst. Figure 2: Stability of the double perovskites under OER conditions. ( a ) OER overpotential measured on the Ir DPs after 1 h of galvanostatic electrolysis plotted as a function of the initial overpotential. ( b ) Evolution of the OER overpotential on Ba 2 PrIrO 6 , Ba 2 YIrO 6 DPs and IrO 2 nanoparticles during 1 h of galvanostatic electrolysis. Full size image The results in Fig. 2a show that Ba 2 PrIrO 6 and Ba 2 YIrO 6 DPs are electrochemically stable on the time scale of 1 h, operating at 10 mA cm −2 , and they show a very similar stability to IrO 2 under the same conditions, which is the state-of-the-art catalyst for OER in acid. The electrochemical stability of these compounds is illustrated by a plot of the Ohmic-drop-corrected overpotential as a function of time during the galvanostatic electrolysis ( Fig. 2b ). Ba 2 PrIrO 6 and Ba 2 YIrO 6 in fact show better stability in terms of overpotential than the IrO 2 catalyst. The La, Nd and Tb-containing DPs are also very active towards OER in acid media according to the JCAP benchmarking, but they lose their activity after 1 h of galvanostatic electrolysis ( Fig. 2a ). It should be realized that the JCAP stability test is not a long-term stability test as required for operation in a commercial device, demanding operation for at least 500 h at current densities higher than 1.6 A cm −2 (ref. 7 ). However, it provides a simple and fast method to estimate both the activity and stability of potentially promising OER catalysts without engineering-related considerations. Due to the small amounts of material used in the OER experiments (ca. 2.5 μg), we could not obtain powder XRD after the catalytic reaction. To assess the structural stability of the Ir DPs, Ba 2 PrIrO 6 was examined by transmission electron microscopy (TEM) and XRD after treatment for 48 h in harsh media, namely 0.1 M HClO 4 and 0.1 M HClO 4 +4 M H 2 O 2 . The Ba 2 PrIrO 6 compound was selected for these experiments because it was one of the compounds that showed to be electrochemically stable ( Fig. 2 ). The open-circuit potentials of the Ba 2 PrIrO 6 DP in 0.1 M HClO 4 solution and in 0.1 M HClO 4 +4 M H 2 O 2 solution were measured to be 1.3 and 1.1 V, respectively. Therefore, the characterization of the treated powder in these two solutions should give an indication of the stability of the DP in acid at the onset of the OER. The TEM images in Supplementary Fig. 3 show that the original powder sample of Ba 2 PrIrO 6 DP consists of rather large particles (ca. 0.5–2 μm), consistent with the sharp lines in the XRD pattern ( Supplementary Fig. 1 ). The particle size of the Ba 2 PrIrO 6 did not change significantly after treatment in 0.1 M HClO 4 or 0.1 M HClO 4 +4 M H 2 O 2 ( Supplementary Fig. 3b,c ) and the XRD pattern ( Supplementary Fig. 4 ) remains virtually the same. This shows that the crystal structure of the DP is preserved during the treatment. However, there is a larger fraction of smaller particles (particle size <200 nm) in the samples that were leached compared with the pristine compound (see Supplementary Fig. 3a in comparison with Supplementary Fig. 3b,c ). This suggests that Ba 2 PrIrO 6 either cleaves or partially dissolves during the treatment but this process is slow ( Supplementary Fig. 4 ). We also characterized the surface composition of the pristine and treated Ba 2 PrIrO 6 DP samples by X-ray photoelectron spectroscopy (XPS). The results of this analysis are summarized in Supplementary Fig. 5 and Supplementary Table 2 in the SI. These data indicate that the surface of Ba 2 PrIrO 6 is not stable on the acid and the oxidative treatment. XPS results show surface enrichment in iridium after both treatments of Ba 2 PrIrO 6 , whereas the barium surface contribution reduces ca. three- to fourfold with respect to the pristine compound. The surface apparently enriches in praseodymium on the oxidative treatment (0.1 M HClO 4 +4 M H 2 O 2 ), but this is caused by the formation of a Pr 2 BaO 4 passivation layer over the perovskite particles. For details, see the Supplementary Note 1 . The XPS results show that the surface iridium sites contain a mixture of Ir(IV) and Ir(V), and become enriched in Ir(V) upon the leaching treatments (see Supplementary Fig. 6 and Supplementary Note 1 ). 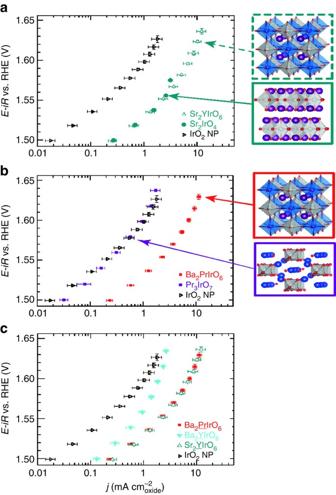Figure 3: Structure sensitivity of the OER activity on the double perovskites. (a) OER activity in 0.1 M HClO4of Sr2YIrO6DP in comparison with Sr2IrO4. (b) OER activity in 0.1 M HClO4of Ba2PrIrO6DP in comparison with Pr3IrO7. (c) Effect of theAandB′cation substitution on the OER activity in 0.1 M HClO4of the Ir DPs. The benchmark activity of IrO2nanoparticles is shown for comparison. Measurements performed under steady-state conditions. The values in the plot are the average of three independent measurements and the error bars correspond to the s.d. The leaching of the components of the Ba 2 PrIrO 6 DP during OER was also assessed by elemental analysis of the electrolyte after electrolysis experiments of 1 h at constant electrode potential ( Supplementary Table 3 ). The post-experiment analysis indicates that ∼ 10 wt% of Ba and Pr leached out of the Ba 2 PrIrO 6 DP in the potential region 1.45–1.55 V, however, a negligible amount of iridium dissolves (<1 wt%), consistent with the evidence from XPS. Role of the crystal structure on the OER activity of Ir DPs The OER activity sensitively depends on the crystal structure of the iridium-based catalyst. Figure 3a,b compares the activity of the Ba 2 PrIrO 6 and Sr 2 YIrO 6 DPs with Sr 2 IrO 4 and Pr 3 IrO 7 phases (the XRD and crystal structure of the Sr 2 IrO 4 and Pr 3 IrO 7 phases are shown in Supplementary Fig. 7 and the XRD of the Sr 2 YIrO 6 is shown in Supplementary Fig. 1 ). The activity of Sr 2 IrO 4 is quite similar to that of Sr 2 YIrO 6 ( Fig. 3a ), whereas that of Pr 3 IrO 7 is 10-fold lower than the Ba 2 PrIrO 6 , though comparable to the activity of the IrO 2 nanoparticles ( Fig. 3b ). The structure of Sr 2 IrO 4 and Pr 3 IrO 7 also contain the corner-shared IrO 6 octahedra, but differ from that of the DP in the network arrangement. The Sr 2 IrO 4 forms two-dimensional (2D) perovskite-like layers [21] , [22] , separated by a rock salt layer of SrO ( Supplementary Fig. 7a ), whereas in Pr 3 IrO 7 the IrO 6 octahedra are linked by sharing the corner oxygen and form one-dimensional (1D) chains [23] ( Supplementary Fig. 7b ). It is important to note that Sr 2 IrO 4 is very unstable under the OER measuring conditions, and its activity abruptly decreases above 1.6 V due to decomposition, hence its OER activity in Fig. 3a is shown until ca. 1.58 V. This illustrates that the 2D arrangement of IrO 6 octahedra is the minimum condition required for the enhanced OER activity but that the activity and stability of the Ir DPs is linked with the 3D perovskite arrangement. Figure 3: Structure sensitivity of the OER activity on the double perovskites. ( a ) OER activity in 0.1 M HClO 4 of Sr 2 YIrO 6 DP in comparison with Sr 2 IrO 4 . ( b ) OER activity in 0.1 M HClO 4 of Ba 2 PrIrO 6 DP in comparison with Pr 3 IrO 7 . ( c ) Effect of the A and B′ cation substitution on the OER activity in 0.1 M HClO 4 of the Ir DPs. The benchmark activity of IrO 2 nanoparticles is shown for comparison. Measurements performed under steady-state conditions. The values in the plot are the average of three independent measurements and the error bars correspond to the s.d. Full size image Regarding the high activity measured for the Ir DPs, we postulate that the crystal lattice strain caused by the small lanthanide and yttrium cations in the B′ site of the DPs may be related to the enhanced OER activity measured in these compounds. DFT calculations have shown that the substitution for small(er) A -site cations can decrease oxygen adsorption energies on simple perovskites ( ABO 3 ), due to the crystal strain [24] . Since IrO 2 has been reported to bind oxygen too strongly for a truly optimal catalyst [25] , [26] , the lattice strain caused by substitution of smaller lanthanides or yttrium could weaken the oxygen adsorption energy and therefore improve the activity of the Ir DPs in comparison with IrO 2 . The effect of strain in the crystal lattice on OER activity of the Ir DPs was further confirmed by comparing the activity measured for Ba 2 YIrO 6 and Sr 2 YIrO 6 ( Fig. 3c ), showing the enhancing effect of the smaller strontium cation on the Ir DP with respect to its barium analogue, in agreement with the computational evidence reported for simple perovskites. The activity of Ba 2 CeIrO 6 shows an additional effect related to the Ir IV centres [12] , [13] ; this increases the binding energy of adsorbates [24] and may explain why this DP is the least active in the series. We speculate that the superior performance of these materials is due to the perovskite-like network optimizing the orbital interaction between the B , B′ cations and O 2− , and allowing adjustment of the B–O and B′–O bond distances to accommodate local charge changes. Since the binding of the OER intermediates requires the iridium centres to adjust their charges, the breathing mode displacement of oxygen in the perovskite-like network would favour lattice adjustments that do not exist in the rutile structure (IrO 2 ) or in fluorite-like compounds. In addition, the observed surface leaching may also contribute to the enhancement of the OER activity of the perovskite surface by leaving behind highly active iridium centres. In summary, we have reported a family of Ir DPs electrocatalysts with superior activity for water oxidation in acid media. Compared with IrO 2 , the state-of-the art benchmarking catalyst, these compounds contain 32 wt% less iridium and exhibit higher activity per real surface area and similar stability for the OER. Our results show that a 3D network of corner-shared octahedra is a necessary prerequisite for the activity enhancement of the Ir DPs as well as for their chemical stability under anodic working conditions. Our findings regarding the effect of the B -site cation on the catalysis towards OER of the Ir DPs suggest that the activity of these compounds might be further improved by carefully selecting the A - and B -site cations. Our strategy for thrifting iridium usage could also be extended to modulate the activity and stability of ruthenium-containing compounds, with a lower content of ruthenium compared with ruthenium oxide. Chemicals The water used to prepare solutions and clean glassware was deionized and ultrafiltrated with a Millipore Milli-Q system (resistivity=18.2 MΩ·cm and TOC<5 p.p.b.). All chemicals used in this work were of high purity (pro analysis grade or superior) and they were used without any further purification. The perchloric acid used for the electrolyte was from Merck (70–72%, EMSURE). Synthesis and characterization of the iridium-based catalysts Ba 2 MIrO 6 (M=La, Ce, Pr, Nd, Tb and Y) double perovskites were prepared from BaCO 3 , SrCO 3 , La 2 O 3 , CeO 2 , Pr 6 O 11 , Nd 2 O 3 , Tb 4 O 7 , Y 2 O 3 and metallic iridium powder, respectively, in alumina crucibles, using the standard solid-state reactions described in literature [13] , [14] , [22] , [23] . All reactions were carried out in air and the products were furnace-cooled to room temperature. The powders were intermittently reground during the synthesis. The suspension of iridium oxide nanoparticles was prepared by acid-catalysed condensation of [Ir(OH) 6 ] 2− intermediate obtained from alkaline hydrolysis of Na 2 IrCl 6 at 90 °C (ref. 27 ). X-ray powder diffraction patterns were collected on a Philips X’Pert diffractometer, equipped with the X’Celerator, using Cu-Kα radiation in steps of 0.020°(2 θ ) with 10 s counting time in the range 10°<2 θ <100°. Electrochemical experiments Glassware was cleaned by boiling in a 3:1 mixture of concentrated sulfuric acid and nitric acid to remove organic contaminants, after which it was boiled five times in water. When not in use, the glassware was stored in a solution of 0.5 M H 2 SO 4 and 1 g l −1 KMnO 4 . To clean the glassware from permanganate solution, it was rinsed thoroughly with water and then immersed in a diluted solution of H 2 SO 4 and H 2 O 2 to remove MnO 2 particles, after which it was rinsed with water again and boiled five times in ultrapure water. The electrochemical experiments were carried out at room temperature in a two-compartment electrochemical cell with the reference electrode separated by a Luggin capillary. Measurements were performed using a homemade rotating Pt ring–Au disk electrode ( φ disk =4.6 mm) as working electrode, a gold spiral as counter electrode and a reversible hydrogen electrode (RHE) as reference electrode; a platinum wire was connected to the reference electrode through a capacitor of 10 μF, acting as a low-pass filter to reduce the noise in the low-current experiments. The electrochemical experiments were controlled with a potentiostat/galvanostat (PGSTAT12, Metrohm-Autolab) and they were performed either with cyclic voltammetry at 0.01 V s −1 or with potentiostatic steps of 0.02 V every 30 s. The latter procedure is referred to as steady-state measurements. Before and between experiments, the working electrode was polished with 0.3 and 0.05 μm alumina paste (Buehler Limited), subsequently it was sonicated in water for 5 min to remove polishing particles. The electrolyte was saturated with air prior to the experiments by bubbling for 20 min with compressed air, with the air first passed through a 6 M KOH washing solution. The RRDE experiments to measure the Faradaic efficiency were carried out with the electrolyte saturated with argon, which was purged through for at least 30 min prior to the experiment and kept passing above the solution during the measurement. For RRDE measurements, the Pt ring was kept at 0.45 V versus RHE while the disk with the catalyst loaded was scanned at 0.01 V s −1 in the potential range 1.25–1.75 V versus RHE. The efficiency ( η ) was calculated with equation (1), assuming that the oxygen reduction proceeds via four electron transfer, to produce water: The collection factor ( N ) for oxygen was measured by using IrO 2 as reference catalyst, and the value obtained was 0.199+0.001, which corresponds well with the value obtained from experiments with the redox couple [Fe(CN) 6 ] 3− /[Fe(CN) 6 ] 4− ( N =0.23); the small difference has been attributed to the non-ideal outward flow of O 2 (ref. 15 ). The catalysts were immobilized on the Au disk by drop-casting an ethanol-based ink of the oxides, using Na-exchanged neutral Nafion as binder [28] . The inks were prepared to yield the following final concentrations: 1 mg oxide /mL ink and 0.7 mg Nafion /mL ink (ref. 29 ). Prior to the preparation, the powders were ground in a mortar to eliminate big clusters. The appropriate amount of ink was drop-cast on the electrode to obtain 15 μg oxide cm disk −2 of loading and this electrode was dried in vacuum; cm disk 2 refers to the geometrical surface area of the Au disk. The current densities reported in this work were calculated using the electrochemical surface area (addressed as real surface area) obtained from pseudo-capacitance measurements, assuming 60 μF cm −2 for the specific capacitance of the double layer [10] , [30] . This procedure of surface area determination was preferred over the Brunauer–Emmet–Teller (BET) method, based on the physical absorption of a gas on the oxide surface, because it allowed us to estimate the active electrochemical surface area in contrast to the surface area obtained from BET measurements [30] . The Tafel plots were corrected for the Ohmic resistance of the electrolyte, the resistance was measured by electrochemical impedance spectroscopy and by conductimetry [10] and the value obtained was 24±1 Ω. The amount of dissolved components from the Ba 2 PrIrO 6 after electrochemical water oxidation experiments in 0.1 M HClO 4 was by means of inductively coupled plasma atomic emission spectroscopy (ICP-AES). These experiments were performed potentiostatically (1 h electrolysis) and in non-rotating conditions, using 10 ml of electrolyte. The double perovskite catalyst was drop-cast on a gold disk (950 μg oxide cm disk −2 of Ba 2 PrIrO 6 ), using an ethanol-based ink similar to the one described for the RRDE experiments but with higher perovskite content (30 mg oxide /mL ink ). The electrolyte was analysed directly in a Varian Vista-MPX CCD Simultaneous ICP-AES. The fraction of dissolved metal (% M leached) was calculated as follows: In this equation, m M (mg)in solution was obtained from the ICP-AES analysis after the electrolysis experiment and m M (mg)drop-cast corresponds to the mass of each component of the Ba 2 PrIrO 6 double perovskite, calculated from its stoichiometry. Data availability All relevant data are available from the authors upon request. How to cite this article: Diaz-Morales, O. et al . Iridium-based double perovskites for efficient water oxidation in acid media. Nat. Commun. 7:12363 doi: 10.1038/ncomms12363 (2016).